Functional anatomy of an allosteric protein Synaptic receptors are allosteric proteins that switch on and off to regulate cell signalling. Here, we use single-channel electrophysiology to measure and map energy changes in the gating conformational change of a nicotinic acetylcholine receptor. Two separated regions in the α -subunits—the transmitter-binding sites and αM2–αM3 linkers in the membrane domain—have the highest ϕ -values (change conformation the earliest), followed by the extracellular domain, most of the membrane domain and the gate. Large gating-energy changes occur at the transmitter-binding sites, α -subunit interfaces, the αM1 helix and the gate. We hypothesize that rearrangements of the linkers trigger the global allosteric transition, and that the hydrophobic gate unlocks in three steps. The mostly local character of side-chain energy changes and the similarly high ϕ -values of separated domains, both with and without ligands, suggest that gating is not strictly a mechanical process initiated by the affinity change for the agonist. Nicotinic acetylcholine receptors (AChRs) are ion channels that generate membrane currents by undergoing a C(losed channel)↔O(pen channel) allosteric transition (‘gating’). AChRs are members of the pentameric ligand-gated ion channel (pLGIC) family whose members include neurotransmitter receptors and prokaryote homologues that respond to pH or extracellular ligands [1] . Here we probe the mechanism of the global, gating conformational change of a muscle AChR by mapping side-chain energy parameters onto X-ray structures of homopentameric pLGICs in non-conducting and ion-conducting conformations [2] , [3] , [4] , [5] , [6] . The adult neuromuscular AChR is a heteropentamer, with 2 α (1)-, β- , δ- and ε -subunits arranged around a central pore ( Fig. 1a ). The extracellular domain (ECD) of each subunit is mostly a β -barrel with connecting loops and the transmembrane domain (TMD) is mostly a four-helix bundle (M1–M4) [7] . The interface between the ECD and TMD has little secondary structure and comprises mainly of loops, including an important linker that connects the M2 and M3 helices. In prokaryote pLGICs, opposing twists of the ECD and TMD, a radial bend of M2, unpacking of the membrane helix bundle and the disruption of barriers to ion permeation are apparent structural correlates of the C→O transition [1] . 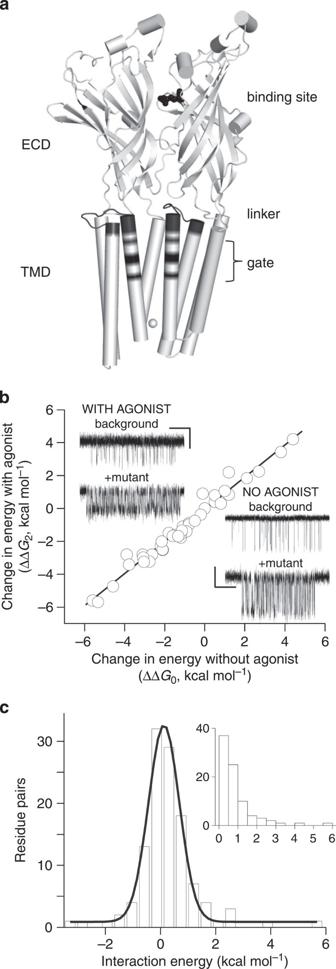Figure 1: Structure and function. (a) Cartoon showing two of the five GLIC subunits. The extracellular and transmembrane domains are labelled (ECD and TMD) along with three functionally important regions in AChRs (the transmitter-binding site, the gating linker and the M2 gate region). White sphere at bottom is Na+. (b) In AChRs, the effect of a mutation on the energy difference between the gating end states (C and O) is approximately the same with or without agonists at the transmitter-binding sites (seeSupplementary Fig. S1). Each circle is a different mutation (Supplementary Table S1). Inset: single-channel currents showing the effect of one mutation (αN217T, in M1) relative to the background (Open is down; scale bar, 0.2 s, 2 pA with or 7 pA without agonist). Energies were estimated from the current interval durations. The diliganded current amplitude is smaller because of fast channel block by the agonist (choline). (c) Interaction energies from mutant cycle analyses (86 pairs)14,30,42,43,44,45. The interaction energy is the difference between the energy change caused in the double mutant versus the sum of the effects for each mutation alone. On average, the interaction energy between separated residues is small but the width of the distribution suggests that there is some energy coupling over distance. Large interaction energies are from neighbors that share a common C versus O environment. Inset, absolute values of the interaction energies (median, 0.6). Figure 1: Structure and function. ( a ) Cartoon showing two of the five GLIC subunits. The extracellular and transmembrane domains are labelled (ECD and TMD) along with three functionally important regions in AChRs (the transmitter-binding site, the gating linker and the M2 gate region). White sphere at bottom is Na + . ( b ) In AChRs, the effect of a mutation on the energy difference between the gating end states (C and O) is approximately the same with or without agonists at the transmitter-binding sites (see Supplementary Fig. S1 ). Each circle is a different mutation ( Supplementary Table S1 ). Inset: single-channel currents showing the effect of one mutation (αN217T, in M1) relative to the background (Open is down; scale bar, 0.2 s, 2 pA with or 7 pA without agonist). Energies were estimated from the current interval durations. The diliganded current amplitude is smaller because of fast channel block by the agonist (choline). ( c ) Interaction energies from mutant cycle analyses (86 pairs) [14] , [30] , [42] , [43] , [44] , [45] . The interaction energy is the difference between the energy change caused in the double mutant versus the sum of the effects for each mutation alone. On average, the interaction energy between separated residues is small but the width of the distribution suggests that there is some energy coupling over distance. Large interaction energies are from neighbors that share a common C versus O environment. Inset, absolute values of the interaction energies (median, 0.6). Full size image Each adult neuromuscular mouse AChR has two functionally equivalent neurotransmitter-binding sites in the ECD, at α – ε and α – δ subunit interfaces. The allosteric gating transition occurs both with and without agonist molecules present at these sites [8] , [9] . Without agonists, the C↔O equilibrium constant is small (~7.4 × 10 −7 ) and there is essentially no resting current [10] . An acetylcholine (ACh) molecule at either binding site increases this equilibrium constant by a factor of ~6,000, so that when both sites are filled the probability of being Open is ~1. The global gating conformational change of the ~300 kDa AChR complex occurs on the ~μs timescale. One way to peer inside a fast chemical reaction is by ϕ -value analysis [11] . AChR gating appears as a one-step, all-or-none reaction in our experiments. However, such a global switch in conformation is a priori that comprises many microscopic rearrangements, each with a corresponding energy change. These events are too brief to be resolved directly by using electrophysiology. Our approach to dissecting the events within AChR gating is to substitute side chains and measure changes in C↔O rate and equilibrium constants estimated from single-channel current interval durations ( Fig. 1b , insert). By taking the logarithms of these constants, we gained estimates of the relative progress of side-chain energy changes within the gating transition state ensemble (TSE; ϕ ), as well as the range of mutational free-energy changes between the two ground states. Below, we colour structures (computed from diffraction patterns) by energies (computed from rate constants) to deconstruct the blur that is AChR gating. We observe that mutations cause mostly local energy changes. There are five ϕ -groups, with residues from each group clustered in the protein along a decreasing gradient between the binding sites and the gate. The transmitter-binding sites and linkers in the α -subunit membrane domain, however, have similarly high ϕ -values even though these regions are separated by ~3 nm. This suggests that these two distant domains do not interact with each other by a mechanical process. Energy measurements In AChRs, most of the gating energy change caused by a side-chain substitution can usually be pinpointed to the location of the mutated amino acid [12] . Mutations away from the binding site only affect the intrinsic C↔O equilibrium and have little or no effect on the energy from the agonist affinity change and vice versa ( Fig. 1b , Supplementary Table S1 and Supplementary Fig. S1 ) [9] . This suggests that the affinity for the transmitter is determined mainly by local interactions at the binding sites. In addition, most mutational effects on gating are nearly independent of each other ( Fig. 1c ). This suggests that little of the energy change associated with a side chain’s gating rearrangement (‘resettling’) is transferred over distance. Third, it is possible to engineer gating rate and equilibrium constants by combining background mutations, voltage and agonists [13] . This ability to design and control the AChR-gating response is a strong confirmation that most mutations affect only the allosteric constant (the unliganded O versus C energy) and do so independently of each other. In AChRs, gating-energy changes mainly reflect differences in the local environment between the ground states, with regard to both mutations and agonists. This local-and-independent nature of agonist and side-chain gating energy changes is an approximation. The s.d. of the distribution shown in Fig. 1c (~1.1 kcal mol −1 ) is larger than our energy resolution (~0.3 kcal mol −1 ); thus, there can be some free-energy coupling between distant residues. For instance, prolines at the two widely separated transmitter-binding sites interact by ~0.7 kcal mol −1 (ref. 14 ). Figure 1c (insert) shows the absolute interaction energies for the mutant pairs. The median of this distribution (~0.6 kcal mol −1 ) is smaller than the median absolute resettling energy for the mutations listed in Supplementary Table S2 (~1.7 kcal mol −1 ). It is possible that more substantial, long-distance free-energy interactions exist in AChR gating, but if so, the results so far suggest that they are rare. We made residue-by-residue maps of two energy parameters, ϕ and range. ϕ is the slope of the rate–equilibrium (R–E) relationship, which is a log–log plot of the forward, C→O rate constant versus the C↔O equilibrium constant for a series of mutations of one residue ( Fig. 2a ). This slope gives the relative position in the TSE where the energy of the perturbed amino acid changes from C-like to O-like in the forward reaction, on a scale from 1 to 0 (ref. 15 ). By measuring ϕ -values of many different residues throughout the protein, it is possible to infer the relative progress of side-chain resettling within the gating TSE. To estimate a ϕ -value, several different side chains are substituted at one amino acid position (the backbone is usually not perturbed). The ‘range’ is the log of the ratio of the equilibrium constant extremes for the mutational series [16] . This value (kcal mol −1 ) is an approximate measure of the extent of the C↔O energy change in the local environment. 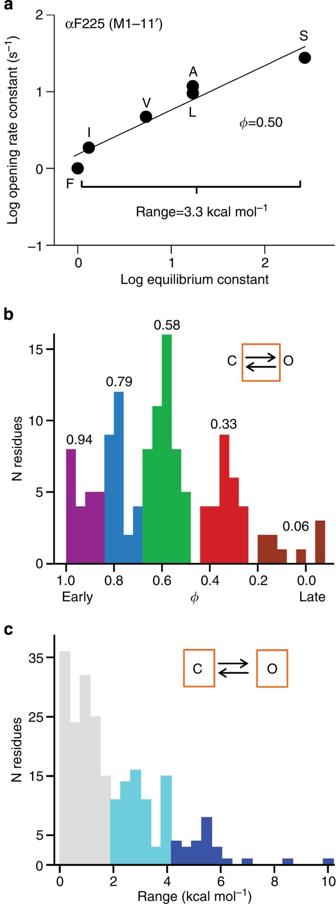Figure 2: Energy parameters (ϕand range). (a) An example R–E plot. Mutations were all of one amino acid (αF225; αM1-15′; seeFig. 7). Each symbol is the mean of ≥3 single-channel measurements for one mutation.ϕis the linear slope and range is proportional to the log of the largest/smallest equilibrium constant ratio. Additional R–E plots are shown inSupplementary Fig. S2. (b) Distribution of AChR gatingϕ-values (Supplementary Table S3).ϕgives the relative position in the forward gating reaction when the residue changes its energy (structure) from C to O. There are five populations: 0.94±0.04 (n=18), 0.79±0.04 (31), 0.58±0.05 (49), 0.33±0.05 (27) and 0.06±0.10 (9) (mean±s.d.). (c) Distribution of range values. Range gives the relative C versus O energy change at the local residue environment. Figure 2: Energy parameters ( ϕ and range). ( a ) An example R–E plot. Mutations were all of one amino acid (αF225; αM1-15′; see Fig. 7 ). Each symbol is the mean of ≥3 single-channel measurements for one mutation. ϕ is the linear slope and range is proportional to the log of the largest/smallest equilibrium constant ratio. Additional R–E plots are shown in Supplementary Fig. S2 . ( b ) Distribution of AChR gating ϕ -values ( Supplementary Table S3 ). ϕ gives the relative position in the forward gating reaction when the residue changes its energy (structure) from C to O. There are five populations: 0.94±0.04 ( n =18), 0.79±0.04 (31), 0.58±0.05 (49), 0.33±0.05 (27) and 0.06±0.10 (9) (mean±s.d.). ( c ) Distribution of range values. Range gives the relative C versus O energy change at the local residue environment. Full size image Here we extend our previous studies and present new ϕ- and range values for 554 mutations of 97 amino acids ( Supplementary Table S2 ). In ~40% of the probed positions, the range was small and a ϕ -value could not be estimated (see Methods). These ‘isoenergetic’ residues may have a ϕ but we could not measure it. An example R–E plot is shown in Fig. 2a and those for the other newly probed positions are shown in Supplementary Fig. S2 . ϕ - and range values for all of the non-isoenergetic AChR residues examined so far are given in Supplementary Table S3 . The combined distribution of ϕ -values for the new residues and those published previously is shown in Fig. 2b . A clustering algorithm was used to determine that there are five ϕ populations with mean values of 0.94, 0.79, 0.58, 0.33 and 0.06. In the ϕ maps, residues are coloured by group, in descending order (purple, blue, green, red and brown, respectively). This colour sequence gives the relative order of reaction progress in channel opening. In the structures, white/beige indicates that a ϕ could not be determined for that position. We also divided the amino acids into three populations and coloured the maps according to range ( Fig. 2c ). Global maps AChR α -subunit ϕ - and range values are mapped onto the full GLIC (presumably Open) pentamer in Figs 3 , 4 , 5 . Although these values for homologous positions in different AChR subunits are sometimes different, it is reasonable to speculate that they may be the same in a homopentamer. The detailed maps of isolated structural domains are shown in Figs 6 , 7 , 8 , 9 , 10 . There are no high-resolution structures of liganded C or O neuromuscular AChRs; hence, our association of AChR energy values with homopentamer structures is provisional. 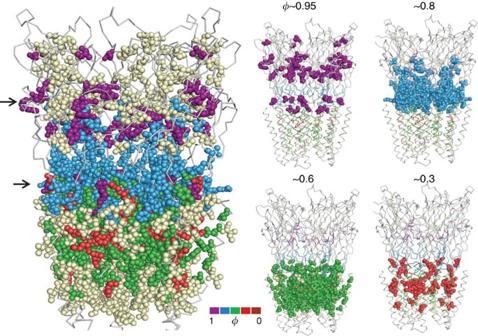Figure 3: AChRα-subunitϕvalues mapped onto the GLIC pentamer. Left, upper and lower arrows mark the level of the transmitter-binding sites and M2–M3 linkers in AChRs. The white ‘isoenergetic’ residues are located mainly above the binding sites and surrounding the TMD (Supplementary Table S3). Right,ϕcolour groups shown individually (seeFig. 2b). There are two, separatedϕ~0.95 (purple) clusters, at the binding sites and the M2–M3 linkers. Theϕ~0.8 (blue; ECD) andϕ~0.6 (green; TMD) residues are tightly clustered, but theϕ~0.3 residues in the TMD are more dispersed. Figure 3: AChR α -subunit ϕ values mapped onto the GLIC pentamer. Left, upper and lower arrows mark the level of the transmitter-binding sites and M2–M3 linkers in AChRs. The white ‘isoenergetic’ residues are located mainly above the binding sites and surrounding the TMD ( Supplementary Table S3 ). Right, ϕ colour groups shown individually (see Fig. 2b ). There are two, separated ϕ ~0.95 (purple) clusters, at the binding sites and the M2–M3 linkers. The ϕ ~0.8 (blue; ECD) and ϕ ~0.6 (green; TMD) residues are tightly clustered, but the ϕ ~0.3 residues in the TMD are more dispersed. 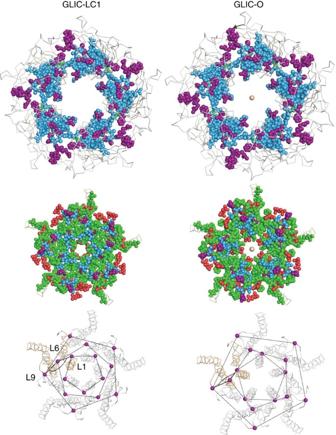Figure 4: AChRα-subunitϕ-values mapped onto non- and ion-conducting GLIC structures. Left, locally closed (LC1) and right, presumably Open (looking down the pore axis from the extracellular compartment). Top and middle, the ECD and TMD (isoenergetic residues not shown). Bottom, the three high-ϕ, purple amino acids in each M2–M3 linker have different configurations in LC1 versus O. Between LC1 and O, the L1–L6–L9 angle changes from ~137° to ~109° (an anticlockwise rotation of L1 and L6 relative to L9) and L1 and L9 are displaced outward by ~25%. Similar comparisons between ELIC and GLIC are inSupplementary Fig. S4. Full size image Figure 4: AChR α -subunit ϕ -values mapped onto non- and ion-conducting GLIC structures. Left, locally closed (LC1) and right, presumably Open (looking down the pore axis from the extracellular compartment). Top and middle, the ECD and TMD (isoenergetic residues not shown). Bottom, the three high- ϕ , purple amino acids in each M2–M3 linker have different configurations in LC1 versus O. Between LC1 and O, the L1–L6–L9 angle changes from ~137° to ~109° (an anticlockwise rotation of L1 and L6 relative to L9) and L1 and L9 are displaced outward by ~25%. Similar comparisons between ELIC and GLIC are in Supplementary Fig. S4 . 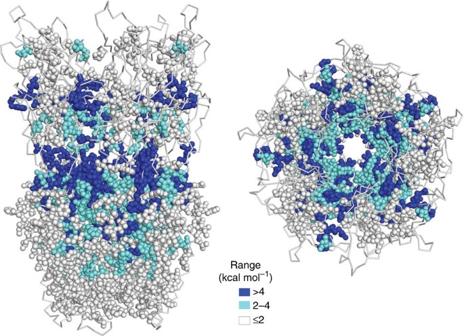Figure 5: AChRα-subunit range values mapped onto the GLIC pentamer. Left, side view and right, top view. Large gating-energy changes are apparent at the binding sites, the ECD–TMD interface, along subunit interfaces, in M1 (seeFig. 7) and in the gate region (seeFig. 8). Full size image Figure 5: AChR α -subunit range values mapped onto the GLIC pentamer. Left, side view and right, top view. Large gating-energy changes are apparent at the binding sites, the ECD–TMD interface, along subunit interfaces, in M1 (see Fig. 7 ) and in the gate region (see Fig. 8 ). 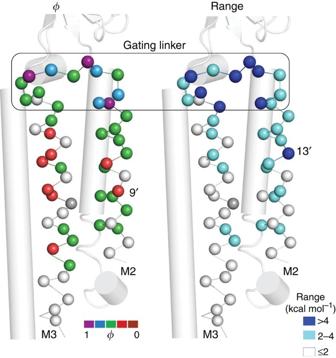Figure 6: Energy maps of αM2–αM3. Only αC atoms are shown (GluCl structure). The top turns of the M2 and M3 helices and the connecting amino acids have largeϕ- and range values (the ‘gating linker’; box). αM2-9′ (left, red) and -13′ (right, navy) are part of a hydrophobic girdle at the gate region (Figs 8cand9). The lipid-facing, red residues in αM3 are at the ivermectin-binding site of GluCl (Supplementary Fig. S3). Full size image Figure 6: Energy maps of αM2–αM3. Only αC atoms are shown (GluCl structure). The top turns of the M2 and M3 helices and the connecting amino acids have large ϕ - and range values (the ‘gating linker’; box). αM2-9′ (left, red) and -13′ (right, navy) are part of a hydrophobic girdle at the gate region ( Figs 8c and 9 ). The lipid-facing, red residues in αM3 are at the ivermectin-binding site of GluCl ( Supplementary Fig. S3 ). 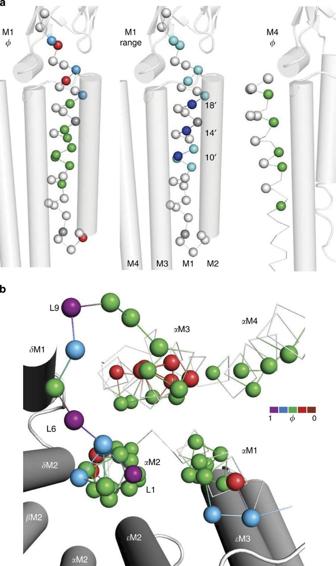Figure 7: Energy maps of αM1, αM4 and the αTMD. In all panels, the structure is GluCl. (a) αM1 and αM4. Left and centre, αM1. The 4′, 10′ and 18′ residues all haveϕ~0.6 and comprise a high-range stripe that faces the helix bundle core (grey, prolines for which aϕcould not be measured). Right,ϕ-values for αM4. Residues that face the core have aϕ~0.6 (green) and those that face the membrane are isoenergetic (white). (b)ϕmap of the αTMD (top view). In allα-subunit TMD helices, most residues that project into the core are green, as are most in all of M2. A cluster ofϕ~0.3 (red) residues in αM3 faces the lipid (seeSupplementary Fig. S3). The fiveϕ~0.8 (blue) residues are all close to the ECD–TMD interface. There are threeϕ~0.95 (purple) residues in the gating linker (L1, L6 and L9). The isoenergetic residues are not shown. Full size image Figure 7: Energy maps of αM1, αM4 and the αTMD. In all panels, the structure is GluCl. ( a ) αM1 and αM4. Left and centre, αM1. The 4′, 10′ and 18′ residues all have ϕ ~0.6 and comprise a high-range stripe that faces the helix bundle core (grey, prolines for which a ϕ could not be measured). Right, ϕ -values for αM4. Residues that face the core have a ϕ ~0.6 (green) and those that face the membrane are isoenergetic (white). ( b ) ϕ map of the αTMD (top view). In all α -subunit TMD helices, most residues that project into the core are green, as are most in all of M2. A cluster of ϕ ~0.3 (red) residues in αM3 faces the lipid (see Supplementary Fig. S3 ). The five ϕ ~0.8 (blue) residues are all close to the ECD–TMD interface. There are three ϕ ~0.95 (purple) residues in the gating linker (L1, L6 and L9). The isoenergetic residues are not shown. 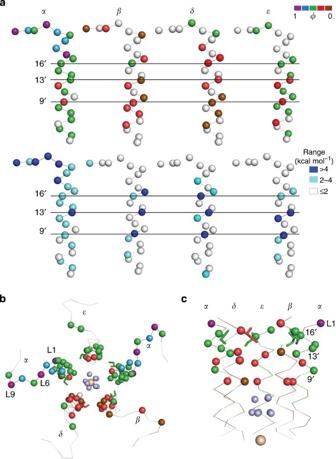Figure 8: Energy maps of M2. In all panels, the structure is GLIC (Open). (a)ϕ(top) and range (bottom) by subunit (2′–26′). The 9′, 13′ and 16′ residues experience large C versus O energy differences (navy). M2 is mostlyϕ~0.6 inαandε, but mostly ≤0.3 inβandδ. The 9′, 13′ and 16′ amino acids are mostly of large range, in all subunits. (b) Top view of the gating linker and M2 showingϕ-values for all AChR subunits (isoenergetic positions not shown). Tan sphere is Na+and light blue spheres are waters. The largeϕand range of the gating linker only pertains to the twoα-subunits. (c) Side view of the gate region. For clarity, only αC atoms of residues with a range ≥3 kcal mol−1are shown. There is a cluster of low-ϕ, high-range residues (9′–16′) above the waters. Full size image Figure 8: Energy maps of M2. In all panels, the structure is GLIC (Open). ( a ) ϕ (top) and range (bottom) by subunit (2′–26′). The 9′, 13′ and 16′ residues experience large C versus O energy differences (navy). M2 is mostly ϕ ~0.6 in α and ε , but mostly ≤0.3 in β and δ . The 9′, 13′ and 16′ amino acids are mostly of large range, in all subunits. ( b ) Top view of the gating linker and M2 showing ϕ -values for all AChR subunits (isoenergetic positions not shown). Tan sphere is Na + and light blue spheres are waters. The large ϕ and range of the gating linker only pertains to the two α -subunits. ( c ) Side view of the gate region. For clarity, only αC atoms of residues with a range ≥3 kcal mol −1 are shown. There is a cluster of low- ϕ , high-range residues (9′–16′) above the waters. 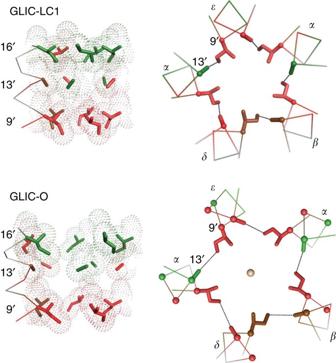Figure 9: Close views ofϕ-values in the M2 gate region. Colour is according toϕ-value (Supplementary Table S3). Left, side view of M2 9′–16′ (extracellular is up). In LC1, the side chains at 16′, 13′ and 9′ form a layered barrier to ion permeation (a gate) that is expanded in O, by energy changes from the green, red and brownϕgroups. The largest ranges in this gate region are at 13′ in all subunits (Fig. 8), perhaps because these side chains are positioned in the middle of the sandwich. Right, top view of the 9′–13′ hydrophobic girdle. α13′ has the highestϕ(0.52, green), and β13′ and δ9′ have the lowestϕ-values (0.12, brown). For the other 9′–12′–13′ positions,ϕ=0.32±0.06 (mean±s.d.;n=9). A similar comparison using ELIC is shown inSupplementary Fig. S4. Full size image Figure 9: Close views of ϕ -values in the M2 gate region. Colour is according to ϕ -value ( Supplementary Table S3 ). Left, side view of M2 9′–16′ (extracellular is up). In LC1, the side chains at 16′, 13′ and 9′ form a layered barrier to ion permeation (a gate) that is expanded in O, by energy changes from the green, red and brown ϕ groups. The largest ranges in this gate region are at 13′ in all subunits ( Fig. 8 ), perhaps because these side chains are positioned in the middle of the sandwich. Right, top view of the 9′–13′ hydrophobic girdle. α13′ has the highest ϕ (0.52, green), and β13′ and δ9′ have the lowest ϕ -values (0.12, brown). For the other 9′–12′–13′ positions, ϕ =0.32±0.06 (mean±s.d. ; n =9). A similar comparison using ELIC is shown in Supplementary Fig. S4 . 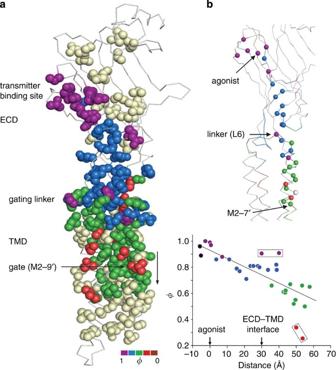Figure 10: AChRα-subunitϕ-values mapped onto a GluCl subunit. (a) Vertical arrow marks the pore. The isoenergetic residues are above the binding sites, below the gate region and facing the membrane. (b) Top,ϕ-values along a pathway that connects the binding site with the gate via loop 2. Bottom, along this structure,ϕdecreases approximately linearly at a rate of 0.063±0.006 nm−1. Boxed, L6 and L1 in the gating linker (purple) and M2-12′ and 9′ in the gate region (red); when these four are included in the linear fit, slope=−0.072±0.01 nm−1. Full size image Figure 10: AChR α -subunit ϕ -values mapped onto a GluCl subunit. ( a ) Vertical arrow marks the pore. The isoenergetic residues are above the binding sites, below the gate region and facing the membrane. ( b ) Top, ϕ -values along a pathway that connects the binding site with the gate via loop 2. Bottom, along this structure, ϕ decreases approximately linearly at a rate of 0.063±0.006 nm −1 . Boxed, L6 and L1 in the gating linker (purple) and M2-12′ and 9′ in the gate region (red); when these four are included in the linear fit, slope=−0.072±0.01 nm −1 . Full size image To a first approximation, there is a top-down, decreasing gradient in ϕ between the binding sites and the gate region ( Figs 3 and 4 ; see also Fig. 10 ). In diliganded gating, residues in the vicinity of the binding sites are mostly purple ( ϕ ~0.95), residues in ECD are mostly blue ( ϕ ~0.8), residues in the TMD are mostly green ( ϕ ~0.6) and those in the hydrophobic gate region are mostly red ( ϕ ~0.3; there are no brown, ϕ ~0.06 residues in the α -subunit). Another basic feature of the map is that residues having similar ϕ -values are clustered. Given the knowledge of a residue’s ϕ colour, there is a high probability that its neighbours will be the same. There are two important exceptions to this pattern. First, there are two high- ϕ (purple) clusters that are separated by ~3 nm, one near the transmitter-binding sites and one in the M2–M3 linkers. So far, no contiguous, high- ϕ connection has been found between these two domains. The ϕ -values for some amino acids in the linkers are as high, or higher, than those at the transmitter-binding sites, which suggests that these regions change energy (structure) at approximately the same position in the gating TSE. For example, gating ϕ -values for the binding site residue αY190 and linker residue αS268 are both ~0.90, both with and without agonists ( Supplementary Fig. S2d ). The similarly high ϕ -values of residues in these two discontinuous domains, regardless of whether or not agonists are present, argues against the hypothesis that energy transfer between the binding sites and the TMD occurs by structural elements pulling, pushing or otherwise perturbing each other mechanically as a consequence of the agonist affinity change. The approximately local character of side-chain energy changes and the high ϕ values of residues at the binding sites and the linkers suggest that the AChR allosteric transition is not purely a cuckoo-clock-like mechanical process that is triggered by the formation of the high-affinity agonist complex. The other exception to the general pattern of the ϕ map is that the low- ϕ , red residues in the TMD are scattered. This incoherence may arise from local, independent energy changes in separated regions rather than from the resettling of a single ϕ block. Supplementary Fig. S3 shows that the red patch of residues in M3 ( Fig. 6 ) corresponds to the ivermectin-binding site in GluCl (ref. 2 ) and that those in M1 ( Fig. 7 ) are near an anaesthetic-binding site in GLIC [17] . We speculate that the low ϕ -values of residues in these two regions reflect delayed resettling of side chains, perhaps caused by a viscous local environment of lipid-filled pockets. It may be that the ϕ - and range values here reflect both side-chain rearrangements and a change in the local O versus C energy of the lipids. Figure 4 compares GLIC ϕ maps in a locally Closed (LC1) versus a presumably Open conformation. ( Supplementary Fig. S4 shows a similar comparison using non-conducting ELIC). Overall, there is a small anticlockwise rotation of the ECD and radial expansions of the TMD ϕ groups between LC1 and O. The different orientations of the αC atoms of the ϕ ~0.95 (purple) residues in the M2–M3 linker are considered further below. Figure 5 shows the pentamer map of range. Many α-subunit residues at the ECD–TMD interface undergo a large resettling energy change in C↔O. In the ECD, there are large energy changes at the transmitter-binding sites and along subunit interfaces, which probably arise from the ECD–TMD twist. In the TMD, there are large energy changes at the M2–M3 linker (see Fig. 6 ), the M1 helix ( Fig. 7 ) and the gate region of the pore ( Fig. 8 ). The low-range isoenergetic residues are mostly above the binding site and enveloping the TMD. These regions may move in the gating isomerization, but they do not experience a significant change in their local energetic environment between C and O. Gating linker Figure 6 shows energy parameter maps for the M2 and M3 helices of the α -subunit. The amino acids located between the tops of these helices have high ϕ -values and experience large ranges. Between αI260 and αI274, three amino acids have a ϕ ~0.95 and seven have a range ≥4 kcal mol −1 . In addition to the linker itself, this region contains the topmost turns of the helices at either end. We call the helix-loop-helix stretch of 15 amino acids that connects αM2 and αM3 the ‘gating linker’ and label its residues L1–L15 ( I VELI P ST S SAVPLI; mouse AChR α -subunit). Positions L1, L6 and L9 (bold) have among the highest ϕ values in the protein [18] . Figure 4 (bottom) shows the αC atoms for the three high- ϕ gating linker amino acids, which comprise a set of nested rings. In GLIC LC1→O, the L9 and L1 positions expand radially (by~25%) but the radius at L6 remains nearly constant (see also Supplementary Fig. S4 ). In the AChR-gating TSE, the energies associated with the expansion of L9 and L1 are more O-like ( ϕ ~0.95) than those of the ECD twist ( ϕ ~0.8) and TMD helix unpacking ( ϕ ~0.6; see below). In the two GLIC structures, there is a flexure of the gating linker that alters the L1–L6–L9 αC angle. Relative to the outer L9 ring, both the inner L1 and middle L6 rings rotate ~20° anticlockwise (in the same direction as the ECD) between LC1 and O. Although L6 is a conserved proline in all pLGICs (αP265 in AChRs), it is unlikely that linker flexure involves a full cis–trans isomerization [19] because it is trans in both GLIC-LC1 and GLIC-O, and because many substitutions here are functional [20] , [21] . The molecular forces behind the expansion and flexing of the gating linker backbone remain to be determined. There is a top-down gradient in range in αM2–αM3 ( Fig. 6a , right). The linkers have a large range, most amino acids in the top halves of the helices are in the 2–4 kcal mol −1 category and most in the bottom are isoenergetic. A notable exception is αM2-13′, which has a large range (5.5 kcal mol −1 ). Figure 7a shows detailed maps of αM1 and αM4. In αM1, most residues are ϕ ~0.6, but near the ECD there are ϕ ~0.8 and ϕ ~0.3 amino acids, side-by-side. Below 5′, most ranges are small; hence, ϕ values could not be determined. There is an isolated, low ϕ -residue in the αM1–αM2 loop. Three αM1 positions (10′, 14′ and 18′) have large ranges. Indeed, the range at αV218 (18′) is the largest observed so far for any residue in the AChR (8.4 kcal mol −1 , which corresponds to a >150,000-fold change in gating equilibrium constant between the A and Y substitutions). These three αM1 side chains comprise a stripe that faces the core of the helix bundle. We speculate that the large ranges of these residues are generated by the unpacking of this core, an event that is energetically about midway through the full C↔O transition ( ϕ ~0.6). αM4 residues that face the interior of the helix bundle are also ϕ ~0.6 (green), whereas those that face the lipid are isoenergetic. None of the αM4 residues had a large range. Figure 7b shows a top view of the α -subunit TMD. Most of the residues that face the helix bundle core are ϕ ~0.6. The three purple, ϕ ~0.95 residues of the gating linker are apparent, as is the cluster of red, low ϕ -residues in αM3 that face the lipid. Gate region In adult neuromuscular AChRs, the M2 helices from α -, β- , δ- and ε -subunits form the lumen of the transmembrane section of the pore. ϕ- and range values have been reported previously for all M2 residues in the α - (refs 18 , 22 ) and ε -subunits [16] , and for some in β (ref. 23 ) and δ (ref. 24 ). In GLIC-LC1 (for ELIC, see Supplementary Fig. S4 ), the M2-9′–13′–16′ side chains together comprise a barrier to ion permeation (a gate) [5] , [6] . These side chains are more loosely packed in GLIC-O compared with that in GLIC-LC1, to allow ion conduction. To further explore this functionally important region, we measured ϕ - and range values for all residues between M2-2′ and -27′ in the AChR β -subunit and the unprobed positions in δ . Residues in the gating linker with high ϕ - and large-range value are present only in the α -subunits ( Fig. 8a , top). Most amino acids in this linker of non- α -subunits are isoenergetic. M2 is mostly ϕ ~0.6 (green) in α and ε , but many residues in β and δ have a ϕ ≤0.3 (red or brown). In all subunits, residues at 9′, 13′ and 16′ have a range ≥2 kcal mol −1 ( Fig. 8a , bottom). A top view of the pore ( Fig. 8b ) highlights the high ϕ -values only of the α -subunit gating linkers and the low ϕ -values in β and δ M2. Figure 8c shows a side view of M2 (2′–18′). The 16′ gate position is ϕ ~0.6 in α , β and ε , but only ~0.3 in δ . Most residues between 16′ and a cluster of waters at ~6′ have low ϕ -values. The M2-9′ and -13′ side chains from adjacent subunits interact to form a hydrophobic girdle that is expanded in GLIC-O versus -LC1 ( Fig. 9 ). The ϕ -values for these positions suggest that gate expansion occurs in three steps, either sequentially or by different reaction pathways (see Discussion). The highest- ϕ girdle position is α13′ (green, ϕ =0.52) and the lowest are β13′and δ9′ (brown, ϕ ~0.06). The 9′ and 13′ residues have a large range in all subunits, except α9′. On the basis of the pattern of ϕ and range, gating unlocking appears to involve three sets of energy change. Those of 16′ ( α , β , ε ) and 13′( α ) have the highest ϕ -values, then 13′( δ , ε ) and 9′( α , β , ε ), followed by 13′( β ) and 9′( δ ). The amino terminus of the high- ϕ , α -subunit gating linker is part of the αM2 helix (L1 is αM2 18′); hence, this part of the allosteric transition probably operates by a mechanical linkage. The ϕ ~0.06 (brown) positions are only in the β (26′, 21′, 13′ and 10′) and δ (10′, 9′, 7′ and 5′) subunits ( Fig. 8a ). The ϕ -value at 17′ is smaller in β and δ compared with that in α and ε . Apparently, resettling of the β and δ M2 region is delayed in C→O, more so than in the other subunits. Moreover, the range at β M2-17′ is larger than in the other subunits. ϕ- and range values have been reported previously for many residues in the ECD of the α -subunit (for citations see Supplementary Table S3 ). Figure 10a shows ϕ -values for the entire α -subunit mapped onto GluCl (presumably O). Figure 10b shows ϕ -values along a structural pathway that connects the binding site with the gate via loop 2 (ref. 25 ). Along this track, ϕ declines at a rate of approximately −0.063 nm −1 . The group of blue ( ϕ ~0.8) residues spans the ECD–TMD interface, with no clear discontinuity between loop 2 and the gating linker/M2. The superimposition of AChR gating energy values onto pentameric pLGIC structures is imperfect. The measurements are from different proteins. The spatial resolution of the energy estimates is low (~side chain) and there may be some long-distance coupling between residues. The association of crystal structures with stable functional states is uncertain. Nonetheless, the maps of ϕ and range represent a new way to explore the relationship between structure and function and, hence, the mechanism of an allosteric transition. The key features of ϕ -values for AChR gating are as follows: i ϕ -values range from 1 to 0. In the α -subunit, the smallest value is 0.26±0.04. The ϕ ~0.06 residues are only in β and δ . ii R–E plots are approximately linear. There is no apparent trend for ϕ to decrease as the equilibrium constant increases (Hammond effect [26] , [27] , [28] ). However, as we used background mutations to place the single-channel interval durations within the optimal range for patch-clamp analysis (~0.1–10 ms), the experimental range in equilibrium constant was always ≤3 kcal mol −1 and often smaller than shown in Supplementary Fig. S2 . iii Some of the scatter in the R-E plots can be traced to experimental error, but some likely also arises from small ‘catalytic’ effects of mutations. So far, only one purely catalytic mutant has been identified in AChR gating (αQ48A in loop 2 (ref. 29 )). iv For most positions, gating ϕ -values are the same with or without agonists [9] . However, some amino acids at the binding sites show smaller unliganded ϕ -values [14] , [30] ; so, a residue’s resettling position within the TSE is not absolute. Some ϕ -values are temperature independent [31] . v ϕ -values have a modal distribution. There are five ϕ populations, with the distinction between the purple ( ϕ ~0.95) and blue ( ϕ ~0.8) groups being less sharp than that for the others. vi Residues having similar ϕ -values are clustered. In the α -subunit, the purple (binding site), blue (ECD) and green (TMD) ϕ groups have an approximate dimension of ~30 Å, and the scattered, red groups in the TMD are each ~10 Å. There are a few, isolated amino acids that have ϕ -values different from their neighbours. There are two, separated ϕ ~0.95 domains (binding site and gating linker in the α -subunits). vii ϕ -values in the α -subunit decrease approximately longitudinally between the binding sites and the gate ( Fig. 10b ). Exceptions include the high ϕ (purple)-residues of the gating linker that are sandwiched between the blue and green clusters and low ϕ (red)-residues that are present throughout the TMD. viii The boundaries between ϕ groups are not sharp. All colours are present at the ECD–TMD interface and three are present in the 9′–12′–13′ M2 girdle. Some, but not all, of this blurring may arise from measurement inaccuracies. There are (at least) two fundamentally different ways to rationalize multiple, fractional ϕ -values in an apparently one-step reaction (A 2 C↔A 2 O; Supplementary Fig. S5 ). One is to imagine parallel transition pathways connecting the end states. For example, if there were two energy (structural) paths connecting A 2 C and A 2 O with ϕ -values of 1 and 0, the emergent ϕ in experiments would be the probability that the residue takes the ϕ =1 route. With this model, we interpret the observation that ϕ =0.6 for a green residue in the TMD to indicate that this side chain changes energy by the ϕ =1 path with a 60% probability and by the ϕ =0 path with a 40% probability. It is also possible that the two paths could each have a fractional ϕ , or that there are more than two possible trajectories. There could be five independent paths, with each residue taking the one appropriate to its ϕ -value with a 100% probability. In this model, the ensemble character of the TSE arises from the existence of parallel, alternative gating trajectories. Another view is that multiple, fractional ϕ -values emerge from a single reaction pathway that is populated with metastable intermediates [32] . In this model, the five ϕ populations correspond to five different microscopic transitions arranged in series along a single, broad TSE. Accordingly, purple residues hop over the first microbarrier (to exit C), then blue, green, red and, finally, brown (to enter O). This scheme imposes a relative temporal sequence to the AChR ϕ map with, for example, the blue ECD twist preceding the unpacking of the green TMD helix bundle. Here the ensemble of the TSE is from sequential barriers along a single trajectory. We cannot distinguish these models from experiments that provide only estimates for the overall forward and backward reaction rate constants. All of the above observations regarding ϕ in AChR gating can be rationalized using either a parallel or a serial mechanism. However, some features are more, and others less, consistent with each view. The parallel-path model does not predict a priori a longitudinal gradient in ϕ , or that the tightly packed residues in the hydrophobic girdle should have three different pathway probabilities (or take three different paths). Nonetheless, it is possible that some (unknown) gradient in a physical property (for example, visco-elasticity) exists within the protein to generate the apparent pattern of pathway selection, and that αM2-13′ and εM2-9′ undergo their gating movements by parallel sets of forces. Although the serial mechanism also does not predict a priori a longitudinal gradient in ϕ , such a pattern could emerge if there were some energy transfer between ϕ groups, for example, if the ECD twist increased the probability of TMD helix unpacking. In the sequential scheme, the high- ϕ expansion/flexure of the α -subunit gating linkers (rather than the affinity change at the binding site) appears as the trigger for the overall isomerization, and αM2-13′ acts as a ‘plug’ whose relatively early gating motion allows the girdle to unpack in stages. A potential problem with the simplest serial scheme, in which the microbarriers of the TSE remain constant, is that it predicts more curvature in the R–E plots than is apparent, particularly for the green, ϕ ~0.6 population of residues [33] . On the basis of ϕ alone, it is not possible to make a compelling case for or against either the parallel or serial interpretation of a fractional ϕ -value (specific scenarios for gating by each mechanism are given in Supplementary Fig. 5S ). However, a ~μs gap within open intervals of glycine receptors (an AChR relative) might reflect sojourns in one or more gating intermediate states [34] . If so, this observation would indicate that there is at least one metastable state in at least one gating trajectory. Moreover, the serial and parallel schemes are not mutually exclusive. There could be multiple pathways in AChR gating, some or all of which are populated by metastable intermediate states having <μs lifetimes, too brief to be detected directly by using electrophysiology. Many residues at the α -subunit ECD–TMD interface undergo a large resettling energy change in A 2 C→A 2 O, perhaps caused by the opposing twist that occurs here. In the ECD, there also are large energy changes at the transmitter-binding sites and along subunit interfaces. In the TMD, the largest changes are in the α-subunit gating linkers, αM1 stripe and the hydrophobic gate. All of these side chain-free energy changes, including those associated with the affinity change for the agonist, appear to arise from mostly local resettling events that add approximately independently to set the gating equilibrium constant and do not transfer significant energy over distance. Three of the amino acids in the gating linker have among the highest gating ϕ -values, and others here experience large resettling energy changes, but only in the two α- subunits that house transmitter-binding sites. The expansion and flexure of this linker at the ECD–TMD interface and its high- ϕ , high-range nature, suggest that gating motions here are important. In the serial pathway model for channel opening, the gating linker rearrangement appears to set off the overall channel-opening isomerization, as its energy changes precede those arising from the twists of the ECD and the unpacking of the TMD helix bundle. In AChRs, the linker movements are important energetically only in the two α -subunits (a two-blade propeller), but in homopentamers the linker energy changes are likely to be distributed among all of the subunits (a five-blade propeller). Given the local nature of side-chain energy changes, the existence of two separated high- ϕ regions argues against the view that the affinity change for the agonist initiates the global isomerization. The formation of the high-affinity complex certainly increases the probability that the distant gate is ion conducting, but perhaps only because this event stabilizes O versus C ground state, by local interactions. Low-affinity binding of an agonist to a resting receptor adds a side-chain-sized structural element to a region that mainly comprises loops. We hypothesize that the agonist affinity change increases the probability of being Open simply because when the bound ligand resettles within C→O (much like a side chain), it forms favourable interactions with nearby residues rather than because it starts a mechanical transfer of energy towards the gate. As in all allosteric proteins, sensor (orthosteric) and effector (catalytic) sites must communicate (exchange energy) over distance. An observation that is not explained using either a parallel or a serial gating mechanism is that the high ϕ -residues at the binding sites are apparently coupled to those in the gating linkers. That is, residues in these separated domains either have the same reaction pathway probabilities or move synchronously in channel opening. There is a direct, mechanical linkage between the α -subunit gating linker and the hydrophobic gate, but so far none is apparent between the binding sites and the linker. How do these separated regions communicate? In AChRs, low-affinity agonist binding includes a conformational change at the binding sites [35] and there is much evidence from NMR (nuclear magnetic resonance) studies of other proteins that ligand binding can change backbone entropy at a distance [36] , [37] . The low free energy of the diliganded gating TSE can be attributed to a large entropy [31] . Elastic network models of pLGICs suggest that energy (in the form of vibrational entropy) may be transferred over distance by backbone ‘breathing’ motions [38] , [39] . It is possible that in AChRs allosteric communication starts with low-affinity binding to increase the entropy of the gating linker, via the backbone, outside of the A 2 C↔A 2 O gating transition itself. The modal nature, spatial clustering and longitudinal gradient in ϕ and the detailed energy maps should serve as a framework for understanding the allosteric gating transition of AChRs. Mutagenesis and expression Human embryonic kidney cells (HEK293) cells were maintained at 37 °C (95% air and 5% CO 2 ) and Dulbecco’s minimum essential medium supplemented with 10% (vol/vol) fetal bovine serum plus 1% (vol/vol) penicillin–streptomycin (pH 7.4). Mutations were created using Quik-Change site-directed mutagenesis kit (Stratagene) and confirmed by dideoxy sequencing of the complementaryDNA samples. HEK cells were transiently transfected with a mixture of cDNAs ( α , β , δ , ε , 2:1:1:1 ratio, ~3.5 μg per 35-mm dish) encoding wild-type (WT) or mutant mouse subunits, by calcium phosphate precipitation. cDNA encoding green fluorescent protein (0.1 μg μl −1 per dish) was added as a marker. The cells were washed after ~16 h and electrophysiological recording commenced within 24–48 h. Electrophysiology Single-channel currents were recorded in the cell-attached patch configuration at 23 °C. The bath and pipette solution was PBS containing (mM): 137 NaCl, 0.9 CaCl 2 , 2.7 KCl, 1.5 KH 2 PO 4 , 0.5 MgCl 2 and 8.1 Na 2 HPO 4 (pH 7.4). In liganded experiments, choline (Cho, 20 mM), carbamylcholine (5 mM) or ACh (500 μM) was added to the pipette solution. The pipette potential was held at +70 mV (which corresponds to a membrane potential of approximately −100 mV) in all experiments. The unliganded currents were measured without agonists in the pipette solution. A separate pipette holder was used in these experiments to avoid any contamination from the ligands. Patch pipettes were pulled from borosilicate capillaries to a resistance of ~10 MΩ and coated with Sylgard (Dow Corning). Single-channel currents were recorded using a PC-505B amplifier (Warner Instrument Corp., Hamden, CT) with external low-pass filtering (Warner Instruments, LPF-8) at 20 kHz and digitized at a sampling frequency of 50 kHz using an SCB-68 data acquisition board (National Instruments). Rate constant estimation The single-channel currents were acquired and analysed using QuB software ( www.qub.buffalo.edu ). Both with and without agonists openings were clustered, with intervals within clusters reflecting mostly binding/gating ( Fig. 1b and Supplementary Fig. S1 ) and those between clusters reflecting sojourns in states associated with desensitization. The intracluster currents were idealized into noise-free intervals (after digitally low-pass filtering, 10–15 kHz) by using the segmental k -means algorithm with a two-state, shut↔open model. Rate constants were estimated from the idealized interval durations by using a maximum log-likelihood algorithm after imposing a dead time and correction of 50 μs. Δ G 2 estimation The diliganded forward-opening ( f 2 ) and backward-closing rate constants ( b 2 ) were measured using choline, carbamylcholine or ACh. To insure binding-site saturation, the concentrations used were ~5 times larger than the corresponding resting equilibrium dissociation constants ( K d WT ). The interval durations were usually fitted by a simple two-state scheme to estimate f 2 and b 2 . Sometimes an additional shut state connected was added to accommodate a brief (~2 ms) state associated with desensitization. The diliganded gating free energy (kcal mol −1 ) was calculated as Δ G 2 =−0.59ln( f 2 / b 2 ). Δ G 0 estimation The frequency and clustering of unliganded openings was increased over that of the WT by using a triple mutant background construct α(D97A+Y127F+S269I) (‘DYS’) or βL262S+δL265S. The unliganded forward-opening ( f 0 ) and backward-closing ( b 0 ) rate constants were measured from the single-channel current interval durations. The unliganded gating free energy (kcal mol −1 ) was calculated as Δ G 0 =−0.59ln( f 0 / b 0 ). Background mutations were used to adjust level of constitutive activity to allow the estimation of Δ G 0 for the αS268 mutants ( Supplementary Fig. S2d ). The backgrounds were δI43Q (Glu), αD97A+αY127F (Asp) and αD97A+αY127F+δV269C (Leu). ϕ and range population analysis ϕ -Values ( Fig. 2b and Supplementary Table S3 ) were separated into k -populations by using the segmental k -means algorithm [40] . We tested for all values of k ≤10, using 50 random staring assignments for each k . There was a significant increase in the sum-squared deviation with k ≤5. The range of ϕ within each of the five populations was: purple (≥0.88), blue (0.86–0.71), green (0.67–0.48), red (0.44–0.17) and brown (≤0.15). A similar approach was used to separate ranges into k =3 populations: grey (<2 kcal mol −1 ), cyan (2–4 kcal mol −1 ) and navy (>4 kcal mol −1 ; Fig. 2c ). A ϕ value could not be determined if i) the range was <1.5 kcal mol −1 (‘isoenergetic’), ii) the single-channel kinetics were too complex to allow confident estimation of the gating rate constants or iii) the scatter in the R–E plot was too great (the s.d. of the linear fit was >0.15). Sequence alignment and structures The range and ϕ -values were mapped onto pLGIC structures by using Pymol (Delano Scientific). The structures were of GLIC-Open (accession number 4HFI .pbd) [3] , GLIC-LC1 (accession number 3TLT .pbd) [41] , ELIC (accession number 3RQW .pdb) [4] or GluCl (accession number 3RIF .pdb) [2] . We used the sequence alignment of Hibbs and Gouaux [2] , with the correction suggested by Pan et al. [4] for ELIC. We made mutations in all 15 positions of the α -subunit TMD-gating linker (αI260–αI274). Position αV271 (L12) was isoenergetic; thus, no ϕ -value was estimated. ELIC, GLIC and GluCl only have 14 gating linker amino acids, with the sequence alignment showing a gap at AChR αA270 (L11). In the homopentamer maps, we plotted the ϕ- and range values for αA270 (L11) at the position aligning with αV271 (L12). How to cite this article: Purohit, P. et al. Functional anatomy of an allosteric protein. Nat. Commun. 4:2984 doi: 10.1038/ncomms3984 (2013).